Regulation ofDrosophilacircadian rhythms by miRNA let-7 is mediated by a regulatory cycle MicroRNA-mediated post-transcriptional regulations are increasingly recognized as important components of the circadian rhythm. Here we identify microRNA let-7, part of the Drosophila let-7-Complex, as a regulator of circadian rhythms mediated by a circadian regulatory cycle. Overexpression of let-7 in clock neurons lengthens circadian period and its deletion attenuates the morning activity peak as well as molecular oscillation. Let-7 regulates the circadian rhythm via repression of CLOCKWORK ORANGE (CWO). Conversely, upregulated cwo in cwo- expressing cells can rescue the phenotype of let-7-Complex overexpression. Moreover, circadian prothoracicotropic hormone (PTTH) and CLOCK-regulated 20-OH ecdysteroid signalling contribute to the circadian expression of let-7 through the 20-OH ecdysteroid receptor. Thus, we find a regulatory cycle involving PTTH, a direct target of CLOCK, and PTTH-driven miRNA let-7. Almost all animals display a wide range of circadian rhythms in behaviour and physiology, such as locomotor activity, sleep, learning and memory, mating and endocrine function [1] , [2] , [3] , [4] . The circadian system includes an input pathway, a core clock system and an output pathway [5] . Through the input pathway, a circadian oscillator receives external information, such as light and temperature signals, that entrain the core oscillator [6] . The core clock system is an integrative oscillator for a self-sustaining rhythm, and the output pathways transmit signals from the oscillator to observable rhythms in behaviour and physiology. Numerous studies have focused on the molecular mechanisms and neural network properties of the circadian oscillator. The positive transcriptional regulatory factors CLOCK (CLK) and CYCLE (CYC) form heterodimers that lead to the transcription of the negative regulators PERIOD (PER) and TIMELESS (TIM) via binding to E-boxes in their promoters [7] , [8] . PER and TIM proteins accumulate in the cytoplasm with a delay and enter the nucleus to repress CLK-CYC-mediated transcription by collaborating with other factors like kinases [9] . CLK-CYC also activates two other feedback loops critical for the phase and amplitude of core oscillators and outputs. One feedback loop affecting Clk mRNA cycling is mediated by VRILLE (VRI) and PAR DOMAIN PROTEIN 1 expression [10] , [11] , and another is mediated by CLOCKWORK ORANGE (CWO), which is activated by CLK-CYC [12] , [13] , [14] , [15] . The per and tim genes receive two opposing signals form DNA-binding transcription factors—a direct activation from CLK-CYC and a direct repression from CWO. In addition, CWO regulates the level of the CLK-CYC, presumably through its actions on each of three main loops [16] . So cwo contributes to sustaining a high-amplitude circadian oscillation in vivo [12] , [13] , [14] . The Drosophila rhythm strength is sensitive to the level and timing of cwo expression, although the amplitude of the cwo mRNA oscillation is much weaker than that of the other core clock genes [15] . In the adult fly brain, ~150 clock neurons are organized into six major clusters: three dorsal clusters (DN1, DNs and DN3), a dorsal–lateral cluster and two groups of ventral–lateral neurons (sLNvs and lLNvs) [17] . Under light-dark (LD) conditions, flies show a morning activity peak (M) around the time of lights-on and an evening activity peak (E) around the time of lights-off. Flies can increase their locomotor activity in advance of both dark-to-light and light-to-dark transitions—a phenomenon termed anticipation. The morning and evening anticipatory behaviour is generated in different clusters of clock neurons [18] , [19] . Beyond the abundant information on the transcriptional–translation feedback loops of circadian rhythms, the importance of post-transcriptional mechanisms is increasingly recognized in circadian rhythms [20] , [21] , such as regulation by microRNAs (miRNAs) [22] . The miRNAs are endogenous small non-coding RNAs (19–25 nt) that function in post-transcriptional regulation of gene expression, and are found to target more than 30% of all protein-coding mRNAs in mammals [23] , [24] . Via base-pairing with specific sequences of target genes typically found in mRNA 3′ untranslated regions (3′UTRs), they usually result in gene silencing via translational repression or target mRNA degradation by an RNA-induced silencing complex consisting of Argonaute catalytic subunits (Ago1 in Drosophila ) [25] , [26] . One requirement for specificity is an accurate match between the 5′-proximal ‘seed’ region of the miRNA and the 3′UTRs of its target mRNA [27] . Previous studies have revealed that miRNAs are involved in regulation of the core circadian oscillator and the clock outputs in Drosophila . By immunoprecipitating mRNAs bound to AGO1, Kadener et al. [28] found that core clock genes Clk , Vri and Cwo are associated with RNA-induced silencing complex, and that bantam-dependent regulation of Clk expression is required for circadian rhythm. Two miRNAs (miR-263a and -263b) were also found to exhibit robust daily changes in abundance in wild-type flies that are abolished in the cyc 01 mutants [29] . In addition, the miR-279 influences circadian behavioural outputs via targeting upd , a ligand of the JAK/STAT pathway [30] , and the oscillating miRNA 959–964 cluster impacts Drosophila feeding time and circadian outputs [31] . To further investigate the role of miRNAs in the Drosophila core circadian clock, we focus on the core clock gene cwo because it is rhythmically expressed and contributes to a high-amplitude circadian oscillation of core clock genes in vivo. Drosophila rhythm strength is sensitive to cwo both in expression level and timing [12] , [13] , [14] . Here we report that the miRNA let-7 affects the locomotor rhythm through the circadian-relevant target gene cwo in the central clock. We also study the signal–transduction pathway and molecular mechanism by which let-7 regulates the daily circadian rhythm, and show that let-7 is involved in an ecdysteroid-signalling cycle. Overexpression of let-7 prolongs activity rhythms Because the expression of the let-7 -Complex ( let-7-C ) or let-7 driven by the tim -GAL4 led to embryonic lethality, we used a pdf -Gal4 driver to overexpress let-7-C or let-7 in the pdf -expressing cells (LNvs), which control locomotor activity rhythms. Let-7-C or let-7 overexpression driven by pdf -GAL4 lengthened circadian period about 2 and 1 h, respectively. In flies expressing mutant let-7 ( UAS-mut-let-7 ), which was generated by site-directed mutagenesis of the UAS-let-7 construct, with G-C transitions at seed sequence sites 3-4 of the mature let-7 miRNA and complementary mutations on the opposing side of the hairpin [32] ( Supplementary Fig. 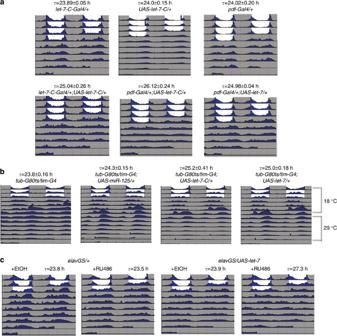Figure 1: Overexpression oflet-7influences locomotor activity rhythms. (a) Overexpression oflet-7-Corlet-7withlet-7-C-Gal4 and pdf-Gal4leads to long behavioural periods in DD. The genotypes are indicated on top of the panels. The white and grey parts indicate light and dark, respectively. (b) Induction oflet-7intimcells leads to long behavioural periods in DD. To restrict expression oflet-7in adults,tim-Gal4-induced expression was repressed during development by atubulin-GAL80ts. Flies were reared and entrained for 3 days following eclosion at 18 °C, free-running activity rhythms were monitored for 3 days at 18 °C, and then the temperature was shifted to 29 °C. The genotypes are indicated on the top of the panels. The white and grey parts indicate light and dark, respectively. (c) Pan-neuronal induction of let-7 in adulthood leads to a long period. Files were reared and then aged for 3 days following eclosion on regular food. They were fed either 500 μMRU486 or ethanol (vehicle control) from the time of entrainment. Average periods of the DD records are shown. The white and gray parts indicate day and night, respectively. Each experiment was conducted at least three times, and 60–90 flies of each genotype were used for behavior assays. 1a ), the circadian period was normal ( Table 1 and Fig. 1a ). These results indicate that let-7 affects circadian period. To exclude the possibility that the behavioural phenotype was caused by ectopic induction of let-7 in neurons where it is usually not expressed, we utilized a knock-in Gal4 in the let-7-C locus ( Supplementary Fig. 1b ) [33] to drive expression of let-7-C , and showed the miRNA levels of let-7 , miR-125 and miR-100 were more abundant ( Supplementary Fig. 2a ). Overexpression of let-7-C driven by let-7-C-Gal4 phenocopies the effect driven by pdf-Gal4 ( Fig. 1a and Table 1 ), suggesting that let-7 regulates circadian rhythms in regions of its normal expression. To distinguish effects of let-7 in adult and in developmental processes, we used a temperature-sensitive tubulin-Gal80 ts coupled with the tim-Gal4 driver to overexpress let-7-C , let-7 and miR-125 in adults. Results showed that the miRNA levels of let-7 and miR-125 were more abundant compared to control ( Supplementary Fig. 2b ). Adult-specific overexpression of let-7-C and let-7 in tim cells resulted in longer circadian periods ( Fig. 1b ) and lower percentages of rhythmic flies when flies were shifted from 18 to 29 °C. Circadian behavioural rhythms were present in 58.1% ( τ =25.2 h, n =43) and 77.8% ( τ =25.0 h, n =45) of the let-7-C and let-7 flies, respectively, in constant darkness (DD), while control flies exhibited normal behavioural rhythms (85.1% rhythmic, τ =23.8 h, n =47). By contrast, the flies with miR-125 overexpression and control flies exhibited similar behavioural rhythm (87.8% rhythmic, τ =24.3 h, n =49). The results show that let-7 affects the central clock. We further drove let-7-C expression with a drug (RU486) inducible pan-neuronal driver (elavGeneSwitch; elavGS ), which also lengthened period in DD ( Fig. 1c ). Taken together, all of these results demonstrate that adult-specific overexpression of let-7 in circadian cells lengthens circadian period and reduces rhythmicity. Table 1 Locomotor activity of flies with altered let-7 levels. Full size table Figure 1: Overexpression of let-7 influences locomotor activity rhythms. ( a ) Overexpression of let-7-C or let-7 with let-7-C-Gal4 and pdf-Gal4 leads to long behavioural periods in DD. The genotypes are indicated on top of the panels. The white and grey parts indicate light and dark, respectively. ( b ) Induction of let-7 in tim cells leads to long behavioural periods in DD. To restrict expression of let-7 in adults, tim-Gal4 -induced expression was repressed during development by a tubulin-GAL80 ts . Flies were reared and entrained for 3 days following eclosion at 18 °C, free-running activity rhythms were monitored for 3 days at 18 °C, and then the temperature was shifted to 29 °C. The genotypes are indicated on the top of the panels. The white and grey parts indicate light and dark, respectively. ( c ) Pan-neuronal induction of let-7 in adulthood leads to a long period. Files were reared and then aged for 3 days following eclosion on regular food. They were fed either 500 μ M RU486 or ethanol (vehicle control) from the time of entrainment. Average periods of the DD records are shown. The white and gray parts indicate day and night, respectively. Each experiment was conducted at least three times, and 60–90 flies of each genotype were used for behavior assays. Full size image Let-7 is required for normal circadian rhythms Deletions of the let-7-C and let-7 , miR-125 had been generated by homologous recombination methods [32] , [33] . Single let-7 , miR-125 , miR-100 mutant strains were generated by deletions of rescuing transgenes, in which the expression of let-7 , miR-100 or miR-125 had been separately eliminated, introduced into strains with deletions of the entire endogenous let-7-C locus—named ▵ let-7 ( KO1/GKI;pP{W8,let-7-C ▵ let-7 }/+), ▵ miR-100 ( KO1/GKI;pP{W8,let-7-C ▵ miR-100 }/+) and ▵ miR-125 ( KO1/GKI;pP{W8,let-7-C ▵ miR-125 }/+) ( Supplementary Fig. 1b ) [33] . In this study, PCR and real time quantitative reverse transcriptase PCR analysis were performed to confirm the deletion of the let-7-C locus and individual miRNAs ( Supplementary Fig. 2c,d ). To test whether the let-7 is required for normal circadian rhythmicity, we analysed the locomotor activity in different let-7-C mutants. Results showed that there was no anticipation of lights-on in let-7-C mutants ( KO1/GKI ) under LD, and this phenotype was conspicuously different from that of wild-type and let-7-C mutant heterozygous flies ( KO1 /+ & GKI /+) ( Fig. 2 ). The ▵ miR-100 mutants exhibited normal morning and evening peaks, suggesting that miR-100 was not responsible for the circadian defect. In contrast, ▵ let-7 , miR-125 mutants exhibited severely suppressed morning peaks before light-on. The absence of lights-on anticipation was also observed in ▵ let-7 mutants but not in ▵ miR-125 mutants ( Fig. 2 ), indicating that let-7 is responsible for the circadian defect in morning anticipation in let-7-C mutants, which could be well rescued by UAS-let-7 in pigment dispersing factor (PDF) neurons ( Fig. 2 ). Because the lights-on response in LD can mask some of the clock-driven morning behaviour [34] , the first day of DD after LD entrainment was also assessed, and this analysis confirmed the lack of morning anticipation in the let-7 mutants ( Fig. 2 ). Besides, both let-7-C and ▵ let-7 , miR-125 mutants became largely arrhythmic in DD (both produced about 50% rhythmic flies), indicating that let-7 is also required for robust 24 h free-running rhythms ( Table 1 ). 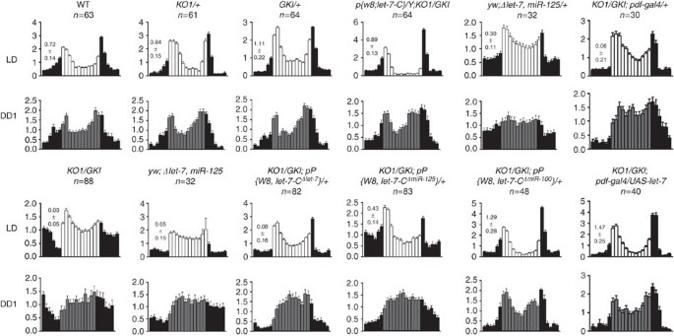Figure 2: Genetic ablation ofLet-7causes flies lose morning anticipation. Comparison of the circadian locomotor activity in light/dark cycles of normallet-7-Cexpression and mutantlet-7-Cexpression flies. Histograms represent the distribution of activity through 24 h, averaged for flies over three LD days and the first day of DD (DD1), and show the activity for each 1 h. Normalized activity profiles are shown. The white and black bars indicate day and night, respectively, while grey and black bars indicate subjective day and night, respectively. Numerical values indicate measures of morning anticipation. Note that genotypes devoid of anticipatory behaviour still respond to light by exhibiting high activity after the light transitions. Total numbers of each genotype are shown in the figure, and each experiment was conducted at least three times. The values were plotted with means±s.e.m. Figure 2: Genetic ablation of Let-7 causes flies lose morning anticipation. Comparison of the circadian locomotor activity in light/dark cycles of normal let-7-C expression and mutant let-7-C expression flies. Histograms represent the distribution of activity through 24 h, averaged for flies over three LD days and the first day of DD (DD1), and show the activity for each 1 h. Normalized activity profiles are shown. The white and black bars indicate day and night, respectively, while grey and black bars indicate subjective day and night, respectively. Numerical values indicate measures of morning anticipation. Note that genotypes devoid of anticipatory behaviour still respond to light by exhibiting high activity after the light transitions. Total numbers of each genotype are shown in the figure, and each experiment was conducted at least three times. The values were plotted with means±s.e.m. Full size image CLOCKWORK ORANGE ( cwo ) is a target of let-7 The Drosophila Cwo gene was identified by bioinformatics as a possible target for let-7 (refs 35 , 36 ) ( Supplementary Fig. 3 ). Cwo produces three mRNAs that encode two different proteins, in which all of the transcripts contain the same ~1.4-kb 3′ UTR. Detection of AGO1-associated mRNAs from fly heads also showed that Cwo might be a miRNA-regulated target [28] . To test whether let-7 can actually regulate the Cwo 3′ UTR, S2 cells were transfected to express the 3′ UTR of Cwo downstream of a luciferase reporter. The cells were also separately transfected to express pri-let-7 (long let-7 precursor). Results showed that the let-7 reduced activity of the luciferase ~70%, and mutation of the let-7 target sites in the seed regions of the Cwo 3′UTR produced a recovery of activity compared to control ( Fig. 3a ). The results in let-7 -transfected S2 cells showed that let-7 expression directly reduced the Cwo mRNA and protein levels ( Fig. 3b ). Moreover, AGO1-associated cwo mRNA from fly heads of wild-type and the ▵ let-7 mutant using the AGO1 IP method of Kadener et al. [28] were also assayed. Results showed that cwo mRNA from AGO1 immunoprecipitates was greatly diminished in ▵ let-7 mutant ( Fig. 3c ). All these results support that cwo is a direct target of let-7. 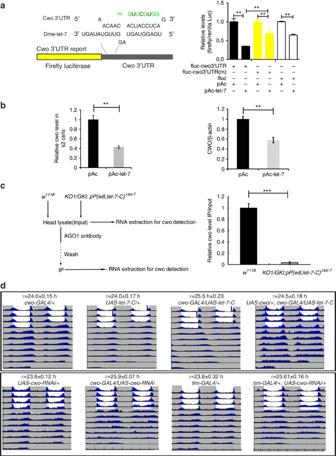Figure 3:Cwois a target oflet-7. (a) The native site of theCwo3′UTR sequence containing thelet-7target was amplified and introduced into a firefly luciferase (fluc) reporter vector (pAc-fluc-cwo3′UTR). Sequence with selected point mutations (m) in theCwo3′UTR was also constructed as a negative control for the same reporter assays. Luciferase reporter assays were performed after cotransfection with pAc-fluc-cwo3′UTR, pAc-fluc-cwo3′UTR (m) or fluc together with an empty vector (pAc) or alet-7expression vector (pAc-let-7). In all cases, cotransfection with pCopia-Renilla Luciferase was performed. For each condition, a normalized firefly/renilla luciferase value was plotted with ±s.e.m. (b)let-7inhibits CWO protein level by affectingCwomRNAin vitro. S2 cells transfected with pAc or pAc-let-7 were lysed and analysed for bothCwomRNA and CWO protein.CwomRNA was detected by quantitative PCR and normalized torp49mRNA, and CWO protein was detected by immunoblot with β-actin as control. Values are reported as fold changes (means±s.e.m.) relative to cells transfected with control expression plasmid. (c) Detection of AGO1-associatedcwomRNAs fromw1118andKO1/GKI;p{w8,let-7-C▵let-7} fly heads. Diagram illustrates the AGO1 IP procedure, and the enrichment ofcwowas calculated as a ratio between the expression values in the immunoprecipitation and the input fractions, normalized to the value forw1118. AGO1-associatedcwomRNA fromw1118was significantly higher than AGO1-associatedcwomRNA fromKO1/GKI;p{w8,let-7-C▵let-7}. (d) Overexpression oflet-7-Cor RNAi knockdown ofcwowithcwo-Gal4ortim-GAL4leads to long behavioural periods in DD. The genotypes are indicated on top of the panels. The white and grey parts indicate light and dark, respectively. Expression ofCwowas able to partially rescue the phenotype oflet-7-Coverexpression incwocells (UAS-cwo/+;cwo-Gal4/UAS-let-7-C) (top panels). Knockdown ofCwoin eithercwo- (bottom panels) ortim-expressing (bottom panels) neurons causes long periods, which mimicked the phenotype oflet-7-Coverexpression. Each experiment was conducted at least three times, and 60–90 flies of each genotype were used for behaviour assays. A significant difference by Student’st-test is indicated (**P≪0.01 and ***P≪0.001). Figure 3: Cwo is a target of let-7 . ( a ) The native site of the Cwo 3′UTR sequence containing the let-7 target was amplified and introduced into a firefly luciferase (fluc) reporter vector (pAc-fluc-cwo3′UTR). Sequence with selected point mutations (m) in the Cwo 3′UTR was also constructed as a negative control for the same reporter assays. Luciferase reporter assays were performed after cotransfection with pAc-fluc-cwo3′UTR, pAc-fluc-cwo3′UTR (m) or fluc together with an empty vector (pAc) or a let-7 expression vector (pAc-let-7). In all cases, cotransfection with pCopia-Renilla Luciferase was performed. For each condition, a normalized firefly/renilla luciferase value was plotted with ±s.e.m. ( b ) let-7 inhibits CWO protein level by affecting Cwo mRNA in vitro . S2 cells transfected with pAc or pAc-let-7 were lysed and analysed for both Cwo mRNA and CWO protein. Cwo mRNA was detected by quantitative PCR and normalized to rp49 mRNA, and CWO protein was detected by immunoblot with β-actin as control. Values are reported as fold changes (means±s.e.m.) relative to cells transfected with control expression plasmid. ( c ) Detection of AGO1-associated cwo mRNAs from w 1118 and KO1/GKI ; p{w8,let-7-C ▵ let-7 } fly heads. Diagram illustrates the AGO1 IP procedure, and the enrichment of cwo was calculated as a ratio between the expression values in the immunoprecipitation and the input fractions, normalized to the value for w 1118 . AGO1-associated cwo mRNA from w 1118 was significantly higher than AGO1-associated cwo mRNA from KO1/GKI ; p{w8,let-7-C ▵ let-7 }. ( d ) Overexpression of let-7-C or RNAi knockdown of cwo with cwo - Gal4 or tim - GAL4 leads to long behavioural periods in DD. The genotypes are indicated on top of the panels. The white and grey parts indicate light and dark, respectively. Expression of Cwo was able to partially rescue the phenotype of let-7-C overexpression in cwo cells ( UAS-cwo /+; cwo - Gal4 / UAS-let-7-C ) (top panels). Knockdown of Cwo in either cwo - (bottom panels) or tim -expressing (bottom panels) neurons causes long periods, which mimicked the phenotype of let-7-C overexpression. Each experiment was conducted at least three times, and 60–90 flies of each genotype were used for behaviour assays. A significant difference by Student’s t -test is indicated (** P ≪ 0.01 and *** P ≪ 0.001). Full size image Does downregulation of Cwo by let-7 contribute to the normal circadian rhythm? To explore this question, we altered the Cwo level by using UAS-let-7-C driven by cwo-GAL4 . Results showed that let-7-C overexpression driven by cwo-GAL4 ( cwo-Gal4/UAS-let-7-C ) lengthened circadian period ( Fig. 3d ), which is consistent with the effect of cwo-RNAi (long circadian period) driven by both cwo - Gal4 and tim - Gal4 ( Fig. 3d ), and it was able to be partially rescued by Cwo overexpression ( UAS -cwo/+; cwo - Gal4 / UAS-let-7-C ) ( Fig. 3d and Supplementary Fig. 4 ). Let-7 expression in cwo neurons ( cwo - Gal4/UAS-let-7 ) resulted in complete lethality. In order to verify that the lethality is due to the reduction of Cwo , we also performed a genetic rescue experiment, in which the viability was normal in UAS-cwo /+; cwo - Gal4/UAS-let-7 transgenic flies compared to controls ( Supplementary Fig. 5 ). Taken together, all these findings demonstrate that miRNA let-7 -mediated Cwo regulation contributes to the circadian rhythm. Let-7 regulates pacemaker neurons Because let-7 appears to function in the central clock, we determined whether let-7 is expressed in the central pacemaker by labelling let-7-C -expressing neurons ( let-7-C - GAL4 × UAS-EGFP ) with green fluorescent protein (GFP) and immunolabeling with anti-PDF antibody. Results showed that let-7 was broadly expressed in the fly brain. The GFP signal was enriched in brain regions such as the mushroom bodies ( Fig. 4a ). The co-detection in brains for GFP and PDF revealed that let-7-C was expressed in the LNvs ( Fig. 4a ). The presence of a GFP signal in clock neurons in let-7-C - GAL4:UAS-EGFP flies further supports the action of let-7 in the central pacemaker. To further investigate the expression of let-7 and its target Cwo in the brain, we also analysed two transcriptional reporters that contain almost the entire first intron of let-7-C ( let-7-Cp12.5kb::lacZ ) or just the 20-OH ecdysteroid (20E)-responsive 3.3 kb fragment ( let-7-Cp3.3kb::lacZ ) with cwo - Gal4 driving GFP [37] . The Cwo reporter was prominently expressed in the LNvs, the PI neurons and the SG ( Fig. 4b ). The spatial expression of lacZ resembled that previously reported in let-7-C - Gal4:UAS-EGFP . All of the reporters exhibit co-expression of let-7-C in the LNv neurons. 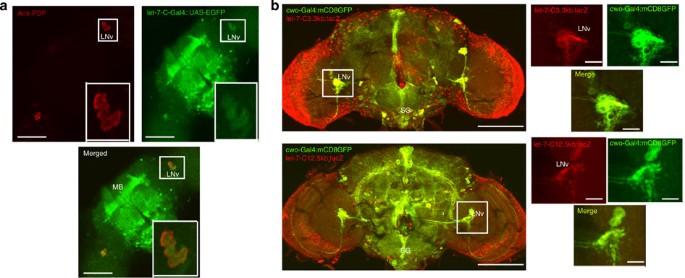Figure 4:let-7is expressed in central clock cells. (a)let-7-C-Gal4is expressed in LNvs. Three- to five-day-old files expressing enhanced green fluorescent protein were entrained to LD for 3 days. Brains were dissected and stained with anti-PDF (red) antibody at ZT1 on the 3rd day in LD, while GFP was detected directly by its fluorescence. The regions in the boxes are magnified in the panels at the bottom right. MB, mushroom bodies. (b)let-7-Cintron 1 transcriptional reporters were used to detectlet-7expression in LNvs. A membrane-targeted mCD8-GFP was expressed inCwoneurons and detectedCwoexpression sites. Brains from the transgenic mutants (cwo-Gal4/UAS-mCD8-GFP;let-7-C3.3kb:lacZ/+ andcwo-Gal4/UAS-mCD8-GFP;let-7-C12.5kb:lacZ/+) were dissected and stained with anti-β-galactosidase at ZT1 on the 3rd day in LD. The region in the box is magnified in the right panels. Each experiment was conducted at least three times, and 10–15 flies of each genotype were used for immunohistochemical assays. Scale bars, 100 μm for the whole-mount figure and 20 μm for the magnified images. Figure 4: let-7 is expressed in central clock cells. ( a ) let-7-C-Gal4 is expressed in LNvs. Three- to five-day-old files expressing enhanced green fluorescent protein were entrained to LD for 3 days. Brains were dissected and stained with anti-PDF (red) antibody at ZT1 on the 3rd day in LD, while GFP was detected directly by its fluorescence. The regions in the boxes are magnified in the panels at the bottom right. MB, mushroom bodies. ( b ) let-7-C intron 1 transcriptional reporters were used to detect let-7 expression in LNvs. A membrane-targeted mCD8-GFP was expressed in Cwo neurons and detected Cwo expression sites. Brains from the transgenic mutants ( cwo-Gal4/UAS-mCD8-GFP;let-7-C3.3kb:lacZ /+ and cwo-Gal4/UAS-mCD8-GFP;let-7-C12.5kb:lacZ /+) were dissected and stained with anti-β-galactosidase at ZT1 on the 3rd day in LD. The region in the box is magnified in the right panels. Each experiment was conducted at least three times, and 10–15 flies of each genotype were used for immunohistochemical assays. Scale bars, 100 μm for the whole-mount figure and 20 μm for the magnified images. Full size image To test whether let-7 affects the central clock, we explored its effects on the daily expression of CWO proteins. Temporal expression profiles of CWO protein in wild-type and let-7-C mutant and ▵ let-7 mutant flies under LD conditions showed that CWO was highly expressed in these two mutant fly heads compared to wild-type flies ( Fig. 5 ). In addition, as shown in Fig. 6 , let-7-C mutant flies and wild-type controls do not exhibit similar daily PER and PDF cycling in the central clock tissue, in which PDF is higher and nuclear PER accumulates sooner in let-7-C mutant flies due to a decrease of let-7 , without an effect on the time of peak nuclear PER accumulation. These results above indicate that let-7 has a function in the core clock through CWO. 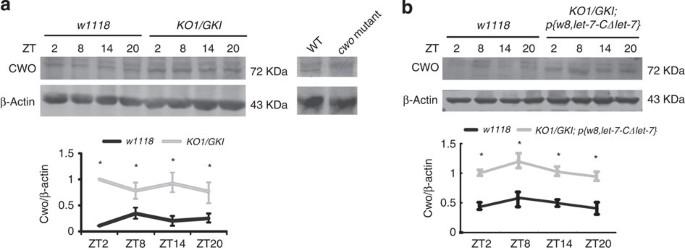Figure 5:let-7affects cwo expression in head. (a) The heads of wild-type (w1118),let-7-Cmutant (KO1/GKI); and (b)▵let-7mutant (KO1/GKI;p{w8,let-7-C▵let-7}; flies were collected at indicated times on the 3rd day of LD. Protein extracts of heads were subjected to western blot analysis using antibodies specific for CWO. β-actin is a loading control. Each experiment was conducted three times, and quantified protein normalized to loading control levels was further normalized to those of the maximum level time point ofKO1/GKIandKO1/GKI;p{w8,let-7-C▵let-7} in each gel. In flies, the homozygousCwomutantscwoe04207were used as control. The quantification curves were plotted as the mean±s.d. of three independent western blots. A significant difference by Student’st-test between wild-type and mutant at the same time point is indicated (*P≪0.05). Figure 5: let-7 affects cwo expression in head. ( a ) The heads of wild-type ( w 1118 ), let-7-C mutant ( KO1/GKI ); and ( b ) ▵ let-7 mutant ( KO1/GKI;p{w8,let-7-C ▵ let-7 }; flies were collected at indicated times on the 3rd day of LD. Protein extracts of heads were subjected to western blot analysis using antibodies specific for CWO. β-actin is a loading control. Each experiment was conducted three times, and quantified protein normalized to loading control levels was further normalized to those of the maximum level time point of KO1/GKI and KO1/GKI;p{w8,let-7-C ▵ let-7 } in each gel. In flies, the homozygous Cwo mutants cwo e04207 were used as control. The quantification curves were plotted as the mean±s.d. of three independent western blots. A significant difference by Student’s t -test between wild-type and mutant at the same time point is indicated (* P ≪ 0.05). 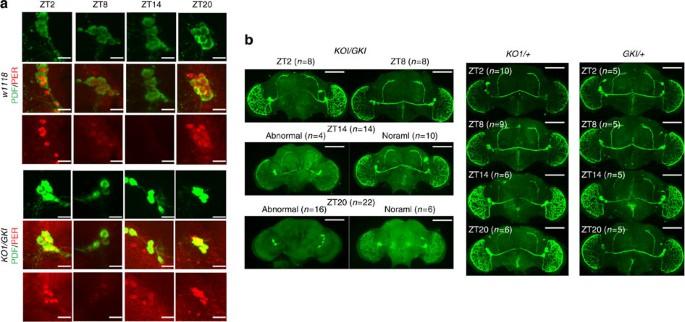Figure 6:let-7-Cmutant flies display abnormal PER and PDF expression. (a)let-7-Cmutant flies show abnormal PER expression in LNvs. The brains of wild-type (w1118) andlet-7-Cmutant (KO1/GKI) flies were collected at the indicated times on the third day of LD and stained with PER (red) and PDF (green) antibodies. (b)let-7-Cmutant flies show abnormal PDF expression in the projections from LNvs. The brains of control heterozygous files (KO1/+ andGKI/+) andlet-7-Cmutant (KO1/GKI) flies were collected at the indicated times on the 3rd day of LD and stained with PDF antibodies. Each experiment was conducted at least three times, and 8–22 flies of each genotype were used for immunohistochemical assays. Scale bars, 100 μm for the whole-mount figure and 20 μm for the magnified images. Full size image Figure 6: let-7-C mutant flies display abnormal PER and PDF expression. ( a ) let-7-C mutant flies show abnormal PER expression in LNvs. The brains of wild-type ( w 1118 ) and let-7-C mutant ( KO1/GKI ) flies were collected at the indicated times on the third day of LD and stained with PER (red) and PDF (green) antibodies. ( b ) let-7-C mutant flies show abnormal PDF expression in the projections from LNvs. The brains of control heterozygous files ( KO1 /+ and GKI /+) and let-7-C mutant ( KO1/GKI ) flies were collected at the indicated times on the 3rd day of LD and stained with PDF antibodies. Each experiment was conducted at least three times, and 8–22 flies of each genotype were used for immunohistochemical assays. Scale bars, 100 μm for the whole-mount figure and 20 μm for the magnified images. Full size image A novel regulatory cycle in circadian rhythm To test whether let-7 itself is regulated by the circadian clock, we further assayed let-7 in wild-type flies and Clk Jrk mutants and found that the expression of mature let-7 exhibited statistically significant (albeit weak) cycling with peak levels in the late day in wild-type flies but not in Clk Jrk flies under an LD condition ( Fig. 7a ). However, pri-let-7-C in wild-type flies did not exhibit a daily rhythm compared to mature let-7 under an LD condition ( Fig. 7a ). This suggests that let-7 cycling may be post-transcriptionally regulated, which is consistent with a previous report [38] . 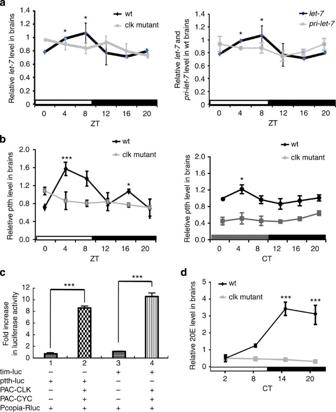Figure 7:Let-7is regulated via PTTH and ecdysteroid signalling. (a) Levels oflet-7are altered inClkJrkmutant flies. Real time quantitative reverse transcriptase PCR analysis of total RNA prepared from adult brains of the indicated genotypes at the indicated time points. The relative expression levels were normalized to 2S RNA levels and were further normalized toClkJrkat ZT0 (left panel). Each time point was compared to ZT0 with Student’st-test. *P≪0.05. The level oflet-7in wild-type fly brains reached a peak in the day but did not inClkJrkflies (left panel). Thepri-let-7-Cdidn’t show oscillation (right panel). (b) Levels ofptthmRNA are altered inClkJrkmutant flies in LD (left panel) and DD (right panel) conditions. The relative expression levels were normalized torp49levels and were further normalized toClkJrkat ZT0. Each time point was compared to ZT0 with Student’st-test. *P≪0.05 and ***P≪0.001. The levels of ptth in wild-type fly brains had rhythmic peaks at ZT4 and ZT16, while they were eliminated inClkJrkflies. (c) Theptthpromoter responds to CLK/CYC. Fold increase in luciferase activity of S2 cells transfected with luciferase reporter constructs containing the promoter ofptthandClk/Cyc-expressing plasmids. Atimpromoter fused to luciferase reporter (tim-luc) was used as positive control. The histogram plot representing fold increase in luciferase activity ±s.e.m. (n=3) is shown. A significant difference with Student’st-test analysis is indicated (***P≪0.001). (d) Levels of 20E are under the control of the central clock. Wild-type andClkJrkmutant fly heads were collected from males at the indicated times for 3 days and 20E levels were measured using radioimmunoassay (RIA). Three experiments with duplicates for each time point were combined and are presented as the mean±s.e.m. The 20E levels at ZT14 and ZT20 were higher than those of other time points by one-way analysis of variance analysis (***P≪0.001). Each experiment was conducted at least three times, and 25–30 fly heads of each genotype were used for the mRNA and RIA detections. Figure 7: Let-7 is regulated via PTTH and ecdysteroid signalling. ( a ) Levels of let-7 are altered in Clk Jrk mutant flies. Real time quantitative reverse transcriptase PCR analysis of total RNA prepared from adult brains of the indicated genotypes at the indicated time points. The relative expression levels were normalized to 2S RNA levels and were further normalized to Clk Jrk at ZT0 (left panel). Each time point was compared to ZT0 with Student’s t -test. * P ≪ 0.05. The level of let-7 in wild-type fly brains reached a peak in the day but did not in Clk Jrk flies (left panel). The pri-let-7-C didn’t show oscillation (right panel). ( b ) Levels of ptth mRNA are altered in Clk Jrk mutant flies in LD (left panel) and DD (right panel) conditions. The relative expression levels were normalized to rp49 levels and were further normalized to Clk Jrk at ZT0. Each time point was compared to ZT0 with Student’s t -test. * P ≪ 0.05 and *** P ≪ 0.001. The levels of ptth in wild-type fly brains had rhythmic peaks at ZT4 and ZT16, while they were eliminated in Clk Jrk flies. ( c ) The ptth promoter responds to CLK/CYC. Fold increase in luciferase activity of S2 cells transfected with luciferase reporter constructs containing the promoter of ptth and Clk/Cyc -expressing plasmids. A tim promoter fused to luciferase reporter (tim-luc) was used as positive control. The histogram plot representing fold increase in luciferase activity ±s.e.m. ( n =3) is shown. A significant difference with Student’s t -test analysis is indicated (*** P ≪ 0.001). ( d ) Levels of 20E are under the control of the central clock. Wild-type and Clk Jrk mutant fly heads were collected from males at the indicated times for 3 days and 20E levels were measured using radioimmunoassay (RIA). Three experiments with duplicates for each time point were combined and are presented as the mean±s.e.m. The 20E levels at ZT14 and ZT20 were higher than those of other time points by one-way analysis of variance analysis (*** P ≪ 0.001). Each experiment was conducted at least three times, and 25–30 fly heads of each genotype were used for the mRNA and RIA detections. Full size image To investigate whether CLK could directly activate let-7 , the let-7-C locus was examined for CLK-biding sites. Since bHLH transcription factors are known to bind to the consensus hexanucleotide sequence E-box (CANNTG) we focused on the various CLK-binding E-boxes described previously [39] . Twenty-one E-boxes were found within a 12.5 kb region surrounding let-7-C . Sixteen of these E-boxes are evolutionarily conserved across five Drosophila genomes ( D.melanogaster , D.simulans , D.sechellia , D.yakuba and D.erecta ). We therefore examined whether CLK-CYC can induce gene expression through these E-boxes in Drosophila S2 cell cultures. Cotransfection with CLK did not induce luciferase expression with 7 fragments from the pri-let-7-C promoter region ( Supplementary Fig. 6 ), indicating that pri-let-7-C cannot be directly regulated by CLK-CYC through E-boxes, and suggesting that the clock regulates let-7 via an indirect pathway. A previous publication has shown that the ecdysteroid receptor (EcR) may effectively target the promoter of let-7-C and activate let-7-C [37] . Thus, it is important to determine if EcR signalling drives let-7-C expression in the adult brain. First, we found that the brain prothoracicotropic hormone (PTTH), an activating hormone for ecdysteroid release, had a daily mRNA rhythm with two peaks at ZT4 and ZT16, and these were blunted in the Clk Jrk mutant in LD ( Fig. 7b ). In addition, the ptth mRNA oscillation in wild-type and Clk Jrk was weakened in DD, although a relatively higher expression at CT4 persisted in wild-type ( Fig. 7b ). The ptth transcriptional periodicity has previously been shown to be correlated with ecdysteroid titre in Drosophila [40] . To further investigate whether CLK could directly activate ptth , we fused the promoter of ptth from the chr2L: 573711–575711 region with luciferase (ptth-luciferase), and then tested it in S2 cells with tim-luciferase as a positive control. Results showed that the ptth-luciferase was significantly activated when co-transfected with CLK/CYC-expressing plasmids ( Fig. 7c ), indicating PTTH is a critical target of the clock and may be involved in regulation of the let-7 oscillation. The most prominent peak of ptth mRNA at ZT 4 is not typical of most CLK/CYC-dependent genes, which peak close to ZT16. However, a previous study showed that PTTH cells might be targets of the s LNv or DN cells and thus stay under control of the master clock [41] . Our results have also shown that ptth is a direct target of CLK/CYC. We speculate that the ZT4 and ZT16 peaks are consequences of multiple circadian inputs to the ptth gene (that is, direct activation by CLK/CYC and inputs resulting from LNv/DN signals). Furthermore, we compared the levels of the 20E steroid hormone (a downstream target of PTTH) at ZT2, 8, 14, 20 between Clk Jrk mutants and wild-type flies, and the results showed that 20E oscillated with a daily rhythm in the wild-type flies but lacked a daily oscillation in the Clk Jrk mutant ( Fig. 7d ). Compared to the 20E oscillation, the oscillation of let-7 showed a significant phase delay ( Fig. 7a,d ). Moreover, a transgenic line in which each of the ecdysone response elements (EcREs) sequences in the let-7-C locus were deleted [37] was used to confirm the necessity of EcREs for circadian let-7-C expression. In contrast to the wild-type lacZ reporter, expression of the mutated let-7-Cp12.5kb ▵ EcRE1-3::lacZ reporter was strongly blocked in the pacemaker neurons ( Fig. 8a ). The ecdysteroid signal is thought to act through a heteromeric receptor composed of the EcR and USP nuclear receptor proteins. So we also blocked ecdysteroid signalling by using the transgenic hs-Gal4-usp.LBD , in which heat shock-induced expression of this USP dominant-negative form disrupts ecdysteroid signalling during adulthood. This resulted in the absence of let-7 oscillations in the fly head and depressed the daytime levels of let-7 ( Fig. 8b ). We further tested the morning and evening peaks of activity in hs-Gal4-usp.LBD flies under LD conditions. Interestingly, we found that adult flies with ecdysteroid-signalling disruption displayed suppressed morning peak anticipation before lights-on ( Fig. 8c ) and became largely arrhythmic in DD ( Supplementary Table 1 ), which mimicked the phenotype of let-7 mutants. Furthermore, lack of 20E signal by inhibiting EcR expression results in decrease of let-7 levels ( Supplementary Fig. 7a ) and increase of Cwo levels ( Supplementary Fig. 7b ), while activation of 20E signal by promoting ptth expression ( Supplementary Fig. 7c ) results in decrease of Cwo levels ( Supplementary Fig. 7d ), and lengthening of circadian period ( Supplementary Fig. 7e ). All of these findings indicate that EcR signalling is required for oscillations of let-7 expression in the fly head and contributes to adult circadian behaviour. 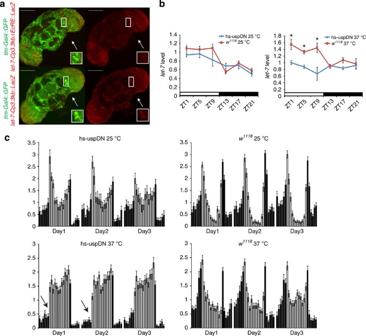Figure 8: Ecdysteroid signalling regulateslet-7and rhythmic behaviour. (a) EcR signalling is required forlet-7-Cexpression in fly heads. The transgenic linelet-7-Cp12.5kb▵EcRE1-3::lacZ37, in which each of the EcREs sequences was deleted, was coupled with atim-Gal4::YFPline to monitor thelet-7expression in clock neurons. In contrast to the wild-type lacZ reporter, expression of the mutated reporter was strongly blocked in the pacemaker neurons. Scale bars, 100 μm for the whole-mount figure. (b) Blocking ecdysteroid signalling affectslet-7circadian expression in heads. Three-day-oldw1118andw1118;hs-Gal4-usp.LBDadult flies were heat shocked (starting from ZT12) at 37 °C for 4 h and allowed to recover to 25 °C for 4 h, and this regime was repeated three times per day for 2 days. After heat shock pulses ended for 12 h, samples (30 heads per each sample) were collected at the indicated time points for RNA extraction and real time quantitative reverse transcriptase PCR analysis. The heat shock method was taken from a reference62with some revision. The relative expression level was plotted as mean±s.e.m. Levels were normalized relative to those ofhs-Gal4-usp.LBDflies seen at ZT1. Thelet-7level at each time point was compared to ZT21 by one-way analysis of variance with Tukeypost-hoctests (*P≪0.05). (c) Blocking ecdysteroid signalling in adult flies results in the loss of the anticipatory morning locomotor activity, thereby mimicking the phenotype oflet-7mutants. The heat shock regime used here was same as that used for panelb. The arrows indicate the loss of the anticipatory morning peaks. Figure 8: Ecdysteroid signalling regulates let-7 and rhythmic behaviour. ( a ) EcR signalling is required for let-7-C expression in fly heads. The transgenic line let-7-Cp12.5kb ▵ EcRE1-3::lacZ [37] , in which each of the EcREs sequences was deleted, was coupled with a tim - Gal4::YFP line to monitor the let-7 expression in clock neurons. In contrast to the wild-type lacZ reporter, expression of the mutated reporter was strongly blocked in the pacemaker neurons. Scale bars, 100 μm for the whole-mount figure. ( b ) Blocking ecdysteroid signalling affects let-7 circadian expression in heads. Three-day-old w 1118 and w 1118 ; hs-Gal4-usp.LBD adult flies were heat shocked (starting from ZT12) at 37 °C for 4 h and allowed to recover to 25 °C for 4 h, and this regime was repeated three times per day for 2 days. After heat shock pulses ended for 12 h, samples (30 heads per each sample) were collected at the indicated time points for RNA extraction and real time quantitative reverse transcriptase PCR analysis. The heat shock method was taken from a reference [62] with some revision. The relative expression level was plotted as mean±s.e.m. Levels were normalized relative to those of hs-Gal4-usp.LBD flies seen at ZT1. The let-7 level at each time point was compared to ZT21 by one-way analysis of variance with Tukey post-hoc tests (* P ≪ 0.05). ( c ) Blocking ecdysteroid signalling in adult flies results in the loss of the anticipatory morning locomotor activity, thereby mimicking the phenotype of let-7 mutants. The heat shock regime used here was same as that used for panel b . The arrows indicate the loss of the anticipatory morning peaks. Full size image From all of these data in this study, we conclude that let-7 functionally regulates circadian rhythm via the core clock component CWO, and we find a novel regulatory cycle for the circadian rhythm mechanism. This cycle is regulated by CLOCK/CYCLE via a pathway involving PTTH, ecdysteroid, its dimeric receptor (EcR/USP), let-7 and CWO ( Fig. 9 ). 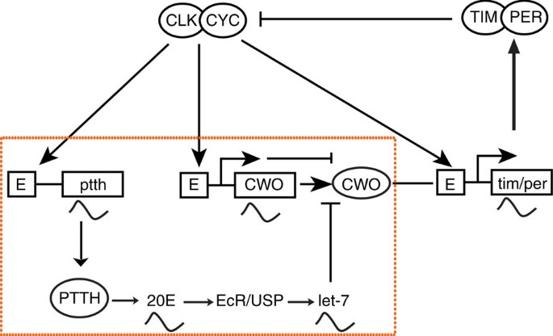Figure 9: A regulatory cycle in the circadian clock. A regulatory cycle for thelet-7pathway (orange dotted line), in whichlet-7functionally regulates circadian rhythm via core clock component CWO, andlet-7is regulated by CLOCK/CYCLE via a pathway involving PTTH, ecdysteroid and its dimer receptor (EcR/USP). The model for CWO downstream effects in the circadian system is adapted from previous studies12,14. Figure 9: A regulatory cycle in the circadian clock. A regulatory cycle for the let-7 pathway (orange dotted line), in which let-7 functionally regulates circadian rhythm via core clock component CWO, and let-7 is regulated by CLOCK/CYCLE via a pathway involving PTTH, ecdysteroid and its dimer receptor (EcR/USP). The model for CWO downstream effects in the circadian system is adapted from previous studies [12] , [14] . Full size image A prior study screened for daily rhythms of miRNAs from wild flies and the mutant cyc 01 by using the microarray method. However, only two Drosophila miRNAs ( miR-263a and miR-263b ) were found to exhibit circadian oscillations [29] . To further investigate miRNAs that exhibit circadian oscillations, Vodala and colleagues used deep sequencing technology to study 18–29 nt RNAs in a 24 h cycle and found a few miRNAs showed significant oscillations. In this study, we found that let-7 showed significant rhythmic oscillation, consistent with the sequencing data from Vodala [31] . However, some miRNAs have been found to play an important role in circadian regulation even though they do not show significant daily oscillations. For example, two important miRNAs ( bantam and miR-279 ) participate in circadian regulation but are not cycling [28] , [30] , [31] . The let-7-C pri-miRNA consisted of miR-100 , let-7 and miR-125 , and these three miRNAs are produced by differential processing in fly heads. Previous studies showed that miR-100 expression was delayed and its expression level was reduced during development compared to let-7 and miR-125 (ref. 37 ). In this study, we found that the expression of pri-let-7-C did not exhibit cycling. However, the expression levels of both the mature let-7 and miR-125 exhibited circadian oscillations, with levels increasing from the late night and reaching a peak in the day, while the miR-100 had no such oscillation ( Fig. 7 and Supplementary Fig. 8 ). Moreover, the expression rhythm of let-7 in the brain is consistent with the expression rhythm of E23—a novel clock gene also induced by ecdyseroid (20E) [42] —and was almost antiphase to that of the 20E. This phase delay is probably due to the time required for post-transcriptional processing of let-7 . It is thought that miRNAs mainly function to fine-tune the levels of key proteins. The miRNAs may have a profound effect on the dynamics of regulatory modules by effects on the amplitude of gene expression and alteration of the frequency in the temporal sequence of gene production or delivery [43] . In this study, we found that the CWO levels were higher in let-7-C null mutant flies ( Fig. 5 ). Additionally, our AGO1 immunoprecipitation in ▵ let-7 showed that cwo is a direct target of let-7 in fly heads ( Fig. 3 ). So let-7 probably contributes to the clock rhythms via regulation of cwo . From our CWO/let-7 co-staining it is clear that both of them are co-present in only some brain cells ( Fig. 4 ). This probably means that the effects on CWO levels observed in let-7 mutants are partially due to expression of both genes in other tissues, such as eyes. Overexpression of CWO in the cwo -expressing cells didn’t generate a let-7 mutant phenotype, but it rescued the rhythm of let-7 overexpression flies ( Fig. 3 ). Moreover, previous studies showed that two copies of Cwo producing overexpression by tim - Gal4 ( tim-Gal4 /+; UAS-cwo ) generate a modest reduction of rhythmic power [12] , [13] , [14] , [15] , which can mimic the let-7 loss–of –function phenotype in this study, indicating that the let-7 mutant phenotype may be due to increased CWO expression. On the contrary, our results show that let-7 overexpression in Cwo cells lengthened circadian period, which is consistent with the effect of cwo-RNAi in both Cwo cells and Tim cells, and it was able to be partially rescued by Cwo overexpression, indicating regulation of Cwo by let-7 . CWO function in regulating expression of per/tim has been clear from previous reports [12] , [13] , [14] , [15] . In this study, results showed that let-7 is expressed in circadian sLNv neurons, behavioural data showed that the fly’s circadian period when let-7-C is overexpressed in endogenous neurons ( let-7-C-Gal4 /+; UAS-let-7-C /+) is longer than wild-type (25.04±0.26), and when it is overexpressed in PDF neurons the period is even longer (26.12±0.24, Table 1 ). The let-7 mutant phenotype is successfully rescued by let-7 re-expression in PDF neuron ( Fig. 2 ). These results suggest that sLNvs are important circadian neurons for regulation of let-7 . Because the UAS-let-7-C seems to have a stronger phenotype that UAS-let-7 , we speculate that three miRNAs ( miR-125 , miR-100 and let-7 ) together may enhance function of let-7 , although miR-125 and miR-100 do not act by themselves. EcR-mediated signalling in the adult fly nervous system is critical for adult behaviour. Immunohistochemical detection showed that EcR was widely expressed in the adult brain [44] . EcR-mediated signalling in adult flies has an important role in the formation of long-term memory) and sleep regulation [44] , [45] , and defective long-term memory and sleep in EcR mutants is thought to be caused by insufficient EcR-mediated signalling. Previous studies showed that deletion of EcREs in the pri-let-7-C locus caused a reduction and delay of let-7-C miRNA expression in adult flies and is associated with a let-7-C mutant phenotype [37] . EcREs in intron 1 of the let-7-C locus play an important role in onset and maintenance of let-7-C expression in a tissue-specific manner [37] . In addition, the let-7-C locus was found to be a direct transcriptional target of 20E because pri-let-7-C RNA could be detected in KC167 cells 30 min after exposure to 20E [37] . Taken together, these data strongly suggest that EcR binds to the endogenous let-7-C locus and activates its transcription in response to 20E, and that this transcriptional regulation is required for miRNA let-7 function [37] . In this study, we showed that CLOCK-PTTH-20E-EcR/USP-mediated signalling contributes to circadian regulation, and 20E mediates circadian expression of let-7 in the adult brain. Moreover, the 20E response is necessary for circadian oscillations in adult pacemaker neurons because the double knockdown of EcR and usp produced an abnormal circadian phenotype [42] . So EcR/USP in circadian neurons receives 20E and mediates the signalling via let-7 , thereby contributing to circadian regulation. However, one complexity to this model is our finding that pri-let-7 mRNA did not exhibit circadian cycling, while let-7 mRNA did cycle. This finding suggests that additional post-transcriptional regulation is necessary to produce cycling of let-7 miRNA, and that pri-let-7 is expressed in additional non-EcR-expressing cells in which it may not be transcribed in a circadian manner and not processed to let-7 (expression in these cells could mask the pri-let-7 oscillation in circadian cells). VRI, a bZIP transcription factor whose expression is controlled by the clock in adult flies [46] , also responds to 20E both in cell culture and in vivo [47] . Interestingly, the ecdysone-signalling pathway was found to function in the adult circadian system; E23—a novel clock gene that encodes the membrane-bound ABC transporter—was induced by ecdysone, and its knockdown in flies increased expression of vri . E23 and vri responded to both ecdysone and clock signals, whereas E23 protein suppressed the ecdysone response and controlled the circadian oscillation through ecdysone-mediated vri expression [42] . The prothoracic gland in Drosophila larvae and pupae, where ecdysone is secreted, is reported to strongly express clock genes [48] , [49] . The rhythmic changes in 20E levels were also regulated by an endogenous circadian oscillator in the haemolymph and testes of adult males in cotton leafworm and in Rhodnius prolixus [50] , [51] , and 20E is also present in Drosophila adults [52] . In this study, we found that the PTTH is a direct target of CLK/CYC, most likely because the 2-kb promoter region of ptth contains 10 noncanonical E-box sequences (CANNTG other than CACGTG). Furthermore, circadian oscillations of PTTH, 20E and let-7 in the brain are caused by CLK. Thus, a novel cycle mediated by ecdysteroid was shown to regulate circadian rhythms in this study. The ultimate target of let-7 miRNA is CWO, and this does not appear to cycle by immunoblot analysis of heads ( Fig. 5 ). However, it is likely that CWO does oscillate in a circadian subset of the cells in which it is expressed, and that constitutive expression in non-circadian cells masks this oscillation in head extracts (note that Fig. 4 shows both let-7 and cwo promoter activity that is more widespread than just circadian cell expression, and Fig. 8 shows that not all let-7 promoter activity is eliminated by deletion of the EcR elements). miRNAs appear to be major players in the regulation of circadian timekeeping. High throughput sequencing experiments have raised the number of miRNAs to 240 in the Drosophila genome [53] . However, only three miRNAs in Drosophila have been clearly reported to function in regulation of circadian rhythm [28] , [30] , [31] . Thus, it may be necessary to perform a genetic screen of individual miRNAs in fly head circadian cells to investigate their potential role in circadian regulation. Recently, a transgenic UAS-miRNA library in Drosophila has been constructed [54] , [55] , [56] . This library circumvents the redundancy issues inherent in loss-of-function screens by facilitating the controlled misexpression of individual miRNAs and is a useful tool to complement loss-of-function approaches. In C.elegans only about 10% of all miRNA deletions had detectable phenotypic consequences, and Schertel et al. [55] validated misexpression as an approach to probe miRNA function. Our analysis of let-7 demonstrates the value of this approach for understanding the role of miRNAs in the fly circadian rhythm. Fly strains Fly strains were maintained on standard molasses-cornmeal-yeast food in a 12 h:12 h LD cycle at 25 °C. The fly lines contain: tim - Gal4 , pdf - Gal4 , cwo - Gal4 , tubulin - Gal80ts , tim - Gal4 , UAS -2x YFP/Cyo , yw , w 1118 , Clk Jrk , hs-Gal4-usp.LBD , UAS-let-7C , UAS-let-7 , UAS-miR-125 , UAS-mut-let-7 , UAS-EGFP , UAS-cwo-RNAi , let-7-C GKI / CyO-TM6b , let-7-C KO1 / CyO-GFP , let-7-C KO1 / CyO;p{w8,let-7-C ▵ let-7 }, let-7-C KO1 ;p{w8,let-7-C ▵ miR-125 }/ CyO-TM6b , let-7-C KO1 / CyO;p{w8,let-7-C ▵ miR-100 }/ TM6b , p{w8,let-7-C 12.5kb::lacZ }, p{w8,let-7- C 3.3kb::lacZ }, p{w8,let-7-C 12.5kb ▵ EcRE::lacZ }. Locomotor behavioural assays Male fly lines were monitored in a 12 h:12 h LD cycle at 25 °C for 3–4 days, followed by 6–7 days in DD using Trikinetics Drosophila Activity Monitors. Activity records were collected in 1 min bins and analysed using Faas (Fly activity analysis suite) software developed by M. Boudinot and derived from the Brandeis Rhythm Package ( http://hawk.bcm.tmc.edu ) described by D. Wheeler [57] . Circadian periods were determined by periodogram analysis [57] . A signal-processing toolbox was used to plot actograms [58] . The morning anticipation was determined by assaying of the locomotor activity [13] . S2 cell culture and luciferase reporter assay The full length 3′UTR of Cwo and an ~500 bp coding region of let-7 (including pre-miR-125 ) were amplified by the PCRusing PrimeSTAR HS DNA Polymerase (TaKaRa). The Cwo 3′UTR was cloned into a pAc5.1-firefly luciferase-V5-His vector and the let-7 coding region was cloned into a pAc5.1-V5-His vector (Invitrogen). The let-7 ‘seed’-targeted sequence in the Cwo 3′UTR was mutated from CTACCTCA to GTTCGTGG using Site-directed, Ligase-Independent Mutagenesis [59] . S2 cells were maintained in 10% fetal bovine serum (HyClone) Schneider’s Insect Medium (Sigma). Cells were seeded in a 12-well plate. Transfection was performed at 70–90% confluence with Cellfectin (Invitrogen) according to the manufacturer’s instructions. In all experiments, 1μg of miRNA expression plasmid, 100 ng of pCopia-Renilla Luciferase and 100 ng of the luciferase firefly reporter were used. Luciferase assays (Dual Luciferase System, Promega) were performed 2 days after transfection. Renilla luciferase activity provided normalization for firefly luciferase activity. AGO1 immunoprecipitation 60 fly heads were homogenized in 700 μl of lysis buffer (30 mM HEPES KOH at pH 7.4, 100 mM KAcetate, 2 mM MgAcetate, 5% glycerol, 0.1% Triton X-100, 1 mM ethylene glycol tetraacetic acid, 5 mM dithiothreitol, 0.4 U μl −1 RNase OUT (Invitrogen), 1 × ethylenediaminetetraacetic acid proteinase inhibitor (Roche)). The lysates were incubated for 10 min on ice and centrifuged at 14,000 r.p.m. for 15 min at 4 °C. One hundred microliters of the supernatant were used as input. To the rest of the supernatant (~500 μl), 1/10 volume of anti-AGO1 antibody (2.0 ug ul −1 , from Miyoshi’s lab) was added and incubated at 4 °C with rotation. After 2 h, 100 μl of protein G plus bead slurry (Invitrogen; previously washed with lysis buffer) was added and incubated for 1 h at 4 °C with rotation. The beads were then recovered by gentle centrifugation. The beads were washed five times (beads plus 500 μl of lysis buffer were rotated for 5 min at 4 °C), before proceeding to RNA extraction. Total RNA from beads of the w 1118 wild-type control and ▵ let-7 mutant ( KO1/GKI;p{w8,let-7-C ▵ let-7} ) at the same circadian time (ZT8) was extracted using Trizol. Real time quantitative reverse transcriptase PCR Flies were collected at the indicated time points and isolated heads were stored at −80 °C. Total RNA (including miRNA) was isolated from 30–50 heads with miRcute miRNA isolation kits (TIANGEN). For reverse transcription and real-time PCR (qRT-PCR) of let-7 , miR-125 , miR-100 and 2s rRNA, we used a miRcute miRNA first-stand cDNA synthesis kit and a miRcute miRNA qPCR detection kit (SYBR Green) (TIANGEN). The miRNA-specific forward primers used for qPCR are shown in Supplementary Table 2 . The reverse primer was a primer complementary to the poly(T) adapter that was provided in the miRcute miRNA qPCR detection kit. For reverse transcription and real-time PCR of Cwo , we used the Quantscript RT kit and RealMasterMix (SYBR Green) (TIANGEN). The sequences of primers are shown in Supplementary Table 2 . All the experiments were performed in the ABI prism 7500 (Applied Biosystems). Western blot analysis Fly heads were homogenized with a pestle, and protein extracts were prepared with radioimmunoprecipitation assay buffer buffer (50 mM Tris–HCl (pH7.4), 150 mM NaCl, 1%NP-40, 0.1% SDS). For immunoblot analysis, proteins were transferred to NC membranes (Pall) and incubated with anti-CWO (1:1,000, from Hardin’s lab) in blocking solution. Band intensity was calculated and analysed with the Gel-Pro Analyzer 4.0. Whole-mount brain immunostaining and microsocopy Adult flies were collected for brain dissection at the indicated times. Brains were fixed for 30–45 min in 4% buffered formaldehyde, washed in phosphate-buffered saline (pH 7.4) with 0.3% Triton X-100 (polybutylene terephthalate), blocked in 5% goat serum in PBT (phosphate-buffered saline tween-20) for 2 h and incubated in primary antibody overnight at 4 °C. Indicated dilutions of the following primary antibodies were made in phosphate-buffered saline tween-20: rabbit anti-PER(1:2,000, from Dr Rosbash), rat anti-PDF (1:2,000 from Dr Ceriani) and rabbit anti-β-galactosidase (1:2,000, Promega). After three 15 min washes, brains were incubated with secondary goat antibodies for 2 h at room temperature, followed by extensive washes. Secondary antibodies included goat anti-rabbit tetramethylrhodamine and goat anti-rabbit fluorescein isothiocyanate. The GFP and yellow fluorescent protein (YFP) were visualized directly by their excitation. All experiments were imaged on a Nikon ECLIPSE TE2000-E and a Nikon D-ECLIPSE confocal microscope (Nikon, Japan). Confocal images were obtained at an optical section thickness of 1–2 μm and finally analysed with Image J. Staining intensity of PER was calculated and normalized as described [60] . 20E quantification To determine the titre of 20E in the heads, we performed a radioimmunoassay developed by David Borst [61] . Briefly, samples were extracted from 50 adult heads by homogenization in 90% methanol. The homogenates were dried at 70 °C using a block heater and then dissolved in 200 μl borate buffer (0.05 M boric acid; 0.9% NaCl; 0.1% gelatin; 0.05% Triton X-100; 7.7 mM NaAzide; pH 8.4) with ~3,000 disintegrations per minute (DPM) [ 3 H]ecdysone and a monoclonal anti-ecdysteroid antibody (diluted 1:12,000). After incubating for 1 h at room temperature and then overnight at 4 °C in the refrigerator, the chilled assay tubes was placed on ice for 5 min, and 500 μl of stirred, cold dextran-coated charcoal was added (2.5 mM boric acid; 0.045% NaCl; 12.5 mg dextran; 38 mM ethylenediaminetetraacetic acid; 7.7 mM NaAzide; 0.5 g charcoal; pH 8.4) to each tube. After 5 min, the samples were centrifuged at 2,000 g for 5 min and the 400 μl supernatant was decanted into a new tube. Two millilitres of scintillation cocktail was added, and the each sample was counted in an LS 6500 scintillation counter (Beckman) for 5 min. Calibration curves were generated using the commercially obtained 20E (Sigma, USA). Statistics analysis Statistical analysis of two data points was performed with Student’s t -test. Statistical analysis of multiple data points was performed with one-way analysis of variance with Tukey post-hoc tests. How to cite this article : Chen, W. et al. Regulation of Drosophila circadian rhythms by miRNA let-7 is mediated by a regulatory cycle. Nat. Commun. 5:5549 doi: 10.1038/ncomms6549 (2014).